Quantitative profiling of peptides from RNAs classified as noncoding Only a small fraction of the mammalian genome codes for messenger RNAs destined to be translated into proteins, and it is generally assumed that a large portion of transcribed sequences—including introns and several classes of noncoding RNAs (ncRNAs)—do not give rise to peptide products. A systematic examination of translation and physiological regulation of ncRNAs has not been conducted. Here we use computational methods to identify the products of non-canonical translation in mouse neurons by analysing unannotated transcripts in combination with proteomic data. This study supports the existence of non-canonical translation products from both intragenic and extragenic genomic regions, including peptides derived from antisense transcripts and introns. Moreover, the studied novel translation products exhibit temporal regulation similar to that of proteins known to be involved in neuronal activity processes. These observations highlight a potentially large and complex set of biologically regulated translational events from transcripts formerly thought to lack coding potential. Recent genome-wide transcriptome studies have shown that tens of thousands of loci outside of the defined protein-coding regions are transcribed [1] , [2] , [3] . The resulting transcripts include a plethora of species such as 5′ leader sequences and 3′ end regions, introns, micro RNAs (miRNAs) [4] , enhancer RNAs [5] , small nuclear RNAs [6] , antisense transcripts [7] , [8] , [9] and various other short and long RNAs [10] . The identification of these transcripts implies a complexity previously unappreciated and has led to the emergence of significant efforts investigating the roles of RNA species traditionally referred to as noncoding sequences [11] , [12] . In parallel to the identification of transcribed regions throughout the genome, proteomic studies have shown that a fraction of the ‘high-quality spectra’ from mass spectrometry (MS)-based experiments do not match annotated proteins [13] . This led us to hypothesize that some of these unmatched spectra could represent uncharacterized translation events derived from transcribed regions outside coding genes. Consistent with this hypothesis, recent studies have shown that noncoding transcripts are associated with ribosome [14] and that some noncoding transcripts lead to translation of short open-reading frames [15] . Here we report the results of a systematic study that we undertook to investigate and evaluate the existence of non-canonical translation products and their biological regulation under physiological conditions combining RNA-seq and quantitative MS approaches. The results of this study not only indicate the presence of a large number of previously undetected protein translational products but they also show that they are temporally regulated, suggesting more complex regulatory biochemical mechanisms that have not been previously observed. Workflow and analysis of RNA-seq data To systematically investigate the existence of non-canonical translation products and their biological regulation under physiological conditions, we introduced and validated new computational algorithms to compare the transcriptome and the proteome from the same experimental context ( Supplementary Fig. 1 ). These algorithms were developed to identify transcripts and corresponding translation products from transcriptome data derived from sequencing total RNA (RNA-sequencing (RNA-seq)), including polyA and non-polyA species, and MS peptide sequencing data. The algorithms were applied to data collected from an experiment in which mouse cortical neurons were depolarized by potassium chloride (KCl) to induce activity-dependent expression changes (see Methods). Total RNA-seq transcriptome data after rRNA depletion [5] and quantitative MS proteomic data were collected at multiple time points ( Fig. 1a ). To identify transcribed regions from the total RNA data, a de novo transcript-calling algorithm was used [16] . This algorithm is well suited to discover unannotated translation products, since it identifies unspliced transcripts, has no sequence biases and is specifically designed to detect lowly expressed regions of the genome. The algorithm identified 26,169 transcribed regions, 12,108 of which overlapped with annotated protein-coding genes (RefSeq, mm9). Here, regions corresponding to unspliced transcripts from total RNA data are searched; thus, our study has the potential to detect a wider range of non-canonical protein products and differs from previous work that was confined to either spliced transcripts [15] or transcripts attached to ribosomes [17] . 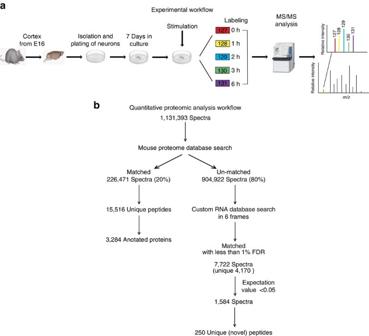Figure 1: Overview of the experimental procedure and peptide identification. (a) Workflow of the KCl depolarization experiment illustrating the collection of total RNA and protein from mouse cortical neurons. Protein samples from multiple time points after depolarization were digested, labelled with isobaric tags and analysed by quantitative proteomic analyses (LC–MS). (b) The resulting spectra were subjected to the database search procedure for filtering and matching peptide spectra. Twenty percent of the spectra matched to the known mouse proteome (Uniprot 12 December 2011, incl. canonical and isoform sequences). The remaining 904,922 spectra were searched against the custom RNA-Seq transcriptome database in six frames and the resulting matched spectra were filtered using stringent criteria as mentioned in the text and of these 250 novel peptides were selected for further analyses. The custom transcriptome was derived from the same samples described. Figure 1: Overview of the experimental procedure and peptide identification. ( a ) Workflow of the KCl depolarization experiment illustrating the collection of total RNA and protein from mouse cortical neurons. Protein samples from multiple time points after depolarization were digested, labelled with isobaric tags and analysed by quantitative proteomic analyses (LC–MS). ( b ) The resulting spectra were subjected to the database search procedure for filtering and matching peptide spectra. Twenty percent of the spectra matched to the known mouse proteome (Uniprot 12 December 2011, incl. canonical and isoform sequences). The remaining 904,922 spectra were searched against the custom RNA-Seq transcriptome database in six frames and the resulting matched spectra were filtered using stringent criteria as mentioned in the text and of these 250 novel peptides were selected for further analyses. The custom transcriptome was derived from the same samples described. Full size image Identification of novel non-canonical translational products A multiplexed quantitative MS proteomic data set comprising three biological replicates with three technical replicates each, with a temporal profile similar to that of the transcriptomic data was acquired and that yielded 1,131,393 MS spectra. We used an iterative procedure to investigate these peptide fragmentation spectra. The rationale for this iterative strategy was to reduce the random matching spectra derived from annotated peptides to non-canonical sequences, thereby increasing the chances of identifying true spectral matches for non-canonical transcripts. First, the spectra were searched with Mascot (v2.3) against an annotated mouse protein database (Uniprot February 2012, canonical and isoform sequences) to identify matches to annotated peptides; 226,471 (20%) of the spectra matched annotated sequences. These matched spectra (peptide spectral matches, PSMs) corresponded to 15,516 unique peptides and were grouped into 3,284 proteins using a 1% false-discovery rate (FDR) cut-off and a minimum of two peptides per protein ( Fig. 1b ). Since the focus in this study was to investigate non-canonical translational events, the spectra matching the annotated proteome were then excluded before searching against the custom transcriptome database. While unmatched good-quality spectra may be derived from peptides that are post-translationally modified and are not accounted for in the initial searches against the canonical mouse protein sequence database, we asked whether some of the unmatched good-quality spectra could constitute translation products from transcripts classified as noncoding RNAs (ncRNAs). To investigate this possibility, the remaining unmatched spectra were searched against a custom database, which was generated by translating the transcribed regions from total RNA-sequence data. This custom database contained transcripts derived from total RNA, including unspliced RNAs and also annotated genes. Each transcript was searched in all six reading frames using Mascot. A 1% FDR was used to select for high-confidence PSMs, resulting in 7,722 PSMs ( Fig. 1b ; of which 54% were non-redundant). To further restrict subsequent analyses to high-quality matches, only the 1,584 matches with a Mascot expectation value <0.05 were chosen for further analysis. The expectation value is equivalent to the E -value in a BLAST search and thus gives each PSM a probability estimate for being a random match. These parameters provide confidence that these hits represent true positives, even though in some cases only a single instance of a peptide is detected [18] . The set of 1,584 PSMs comprised 250 distinct peptides that mapped uniquely to regions of the mouse genome considered noncoding ( Supplementary Table 1 ). 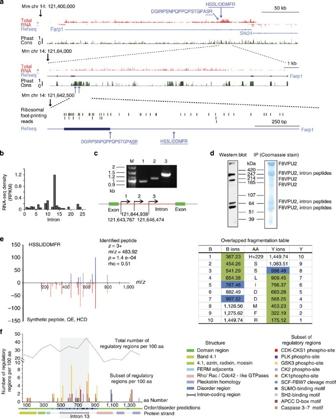Figure 2: Identification and validation of two novel peptides at the FARP1 locus. (a) Screenshot from the UCSC genome browser showing total RNA, ribosomal footprints, Refseq gene structure and degree of conservation (Phast Cons). The bottom part is a zoomed in version spanning intron 13. The arrows indicate the position of the two novel peptides. The first peptide (DGIRPSNPQPPQPSTGPASR) spans an exon–intron boundary; the underlined amino acids are located within the intron. The figure also indicates peptides found from ribosomal footprinting studies. (b) Average read density (RPKM) for all FARP1 introns. (c) RT–PCR gel showing RNA expression of three regions within FARP1 intron from depolarized cortical cells. (d) WB analysis of mouse brain lysate showing FARP1 protein bands of different molecular weights. Coomassie stained SDS–PAGE gel showing IP of FARP1 from mouse brain lysate. The bands were analysed using LC–MS/MS and confirmed as FARP1 (F8VPU2) protein along with peptides from intron (the full gel images ofc,dare inSupplementary Fig. 11). (e) Chemical validation of one of the novel peptides (HSSLIDDMFR) from FARP1 by comparing its spectra with synthetic peptide spectra as described in Methods. The identified peptide (HSSLIDDMFR) spectra (top) and synthetic peptide spectra (bottom) show a strong match with a spearman correlation coefficient (ρ) of 0.51 and a significantPvalue of 1.4e−04. The charge state,m/zvalue,Pvalue and rho value of the peptide are listed. Overlapped fragmentation table indicating the y and b ions that were detected in both ‘identified’ and ‘synthetic’ spectra. The green ions were detected in both spectra, blue were detected only in ‘identified’ spectra. (f) A model showing the domains’, disordered regions’ and regulatory regions’ prediction in FARP1 amino-acid sequence, including the novel coding region of intron 13 by ELM (http://elm.eu.org/). The total number of regulatory regions per 100 amino acids is shown by line graph, out of which the distribution of a subset of functionally important regions per 100 amino acids are indicated by color bars. The number of regulatory regions is enriched in intron 13 coding region. Seven pairs of peptides ( Supplementary Table 2 ) matched two different ncRNAs that differed only by an isobaric I/L amino acid; although the unambiguous identification of the source of these peptides is not possible, it is clear that these peptides sequences are not found in the canonical mouse protein sequences. Given that RNA sequence information was obtained for both I- and L-containing peptides, it is possible that both the I- and the L-containing peptides are present; therefore, all 14 peptides were included for further analysis. Interestingly, both annotated and novel peptides were found for some proteins. For example, the initial database search against the annotated Uniprot database resulted in the identification of nine annotated, unique peptides for Centg2 (Agap1, Supplementary Fig. 2 ) (17% protein sequence coverage), whereas the database search against the custom transcriptome database resulted in the identification of two novel peptides from the first intron of Centg2 (Agap1, Supplementary Fig. 2 ). The 250 high-confidence peptides that were aligned to experimentally defined transcripts are referred to as novel peptides throughout the manuscript ( Fig. 1b ). Evaluation and validation of novel peptides In addition to the high stringency cut-offs used to select peptides, several experiments were performed to evaluate the novelty of the peptides and the validity of the PSMs. First, each of the 250 novel peptide sequences was searched in non-redundant protein sequences from mouse using BLASTP and the UCSC genome browser. The results showed that 31 of the peptides corresponded to either pseudogenes or unannotated genes, which had been predicted to be translated, based on computational and transcriptional evidence, but lacked any supporting protein evidence. None of the remaining 214 peptides showed a similarity to the annotated proteome ( Supplementary Table 1 ). Second, each of the 250 novel peptide sequences was searched against both the peptide atlas ( http://www.peptideatlas.org ) and NIST-Libraries of Peptide Tandem Mass Spectra ( http://peptide.nist.gov ) databases. None of these novel peptides were identified in those databases, confirming that the novel peptides had not been reported in publicly available databases. Third, synthetic peptides were used to chemically validate the identity of the novel peptides. Fragmentation patterns of the synthetic peptides were compared with the mouse peptides identified from the primary data set. This is the most stringent method available for validating an identified peptide, as it constitutes a chemically synthesized positive control. The fragmentation patterns of 45 peptides are presented ( Fig. 2e ; Supplementary Figs 2B, 3, 5B and 7C ). The similarity between the identified and synthetic spectra was evaluated by computing the rank-ordered Spearman correlation coefficient; all the peptides showed strong correlation with a significant P value ( P <0.05). In addition, the average number of common fragment ions identified was greater than 90%. Fourth, the 250 novel peptides were compared against published results from a ribosomal footprinting experiment [14] . Of note, the ribosomal profiling data were performed on mouse embryonic stem cells, which have a different expression profile from mouse neurons. Nonetheless, 34 of the novel peptides were observed to be associated with ribosomes, providing independent evidence consistent with non-canonical translation events. These analyses and validation procedures lend support to the current proof of existence of novel peptides from non-canonical translational events. Figure 2: Identification and validation of two novel peptides at the FARP1 locus. ( a ) Screenshot from the UCSC genome browser showing total RNA, ribosomal footprints, Refseq gene structure and degree of conservation (Phast Cons). The bottom part is a zoomed in version spanning intron 13. The arrows indicate the position of the two novel peptides. The first peptide (DGIRPSNPQPPQPSTGPASR) spans an exon–intron boundary; the underlined amino acids are located within the intron. The figure also indicates peptides found from ribosomal footprinting studies. ( b ) Average read density (RPKM) for all FARP1 introns. ( c ) RT–PCR gel showing RNA expression of three regions within FARP1 intron from depolarized cortical cells. ( d ) WB analysis of mouse brain lysate showing FARP1 protein bands of different molecular weights. Coomassie stained SDS–PAGE gel showing IP of FARP1 from mouse brain lysate. The bands were analysed using LC–MS/MS and confirmed as FARP1 (F8VPU2) protein along with peptides from intron (the full gel images of c , d are in Supplementary Fig. 11 ). ( e ) Chemical validation of one of the novel peptides (HSSLIDDMFR) from FARP1 by comparing its spectra with synthetic peptide spectra as described in Methods. The identified peptide (HSSLIDDMFR) spectra (top) and synthetic peptide spectra (bottom) show a strong match with a spearman correlation coefficient ( ρ ) of 0.51 and a significant P value of 1.4e−04. The charge state, m / z value, P value and rho value of the peptide are listed. Overlapped fragmentation table indicating the y and b ions that were detected in both ‘identified’ and ‘synthetic’ spectra. The green ions were detected in both spectra, blue were detected only in ‘identified’ spectra. ( f ) A model showing the domains’, disordered regions’ and regulatory regions’ prediction in FARP1 amino-acid sequence, including the novel coding region of intron 13 by ELM ( http://elm.eu.org/ ). The total number of regulatory regions per 100 amino acids is shown by line graph, out of which the distribution of a subset of functionally important regions per 100 amino acids are indicated by color bars. The number of regulatory regions is enriched in intron 13 coding region. Full size image Molecular characterization of FARP1 Further in-depth molecular characterization of non-canonical translation was carried out for the FARP1 protein. Two unique novel peptides DGIRPSNPQPPQPSTGPASR and HSSLIDDMR, which were in frame with the rest of the protein, were mapped to the FARP1 intron 13 ( Fig. 2a ). The RNA-seq read density across this intron is approximately tenfold higher than that of the other introns and the RNA levels for this intron are comparable to the levels observed for the exons ( Fig. 2b ). In addition, reverse transcription PCR (RT–PCR) from three regions of this intron showed good expression in cortical cells from same experimental set-up ( Fig. 2c ). Closer inspection of the FARP1 intron 13 sequence reveals that the first 983 bp do not contain a stop codon within the reading frame used by the preceding exon. Thus, we hypothesized that there could be novel isoforms present with ~330 additional amino acids. Western blot (WB) validation was performed to investigate FARP1 (F8VPU2) in brain lysates. FARP1 is FERM, Rho-GEF and pleckstrin domain-containing protein with several different splice variants and varying molecular weights ranging from 51 to 420 kDa ( Fig. 2d ). To validate that FARP1 isoforms are present in the protein bands corresponding to the WBs, an immunoprecipitation (IP) from mouse brain tissue followed by MS analysis was performed. Briefly, when the IP of FARP1 is separated by size on an SDS–polyacrylamide gel electrophoresis (PAGE) gel and stained using Coomassie blue, protein bands are observed at molecular weights ranging from 51 to >420 kDa, as observed from WB results of the whole-cell lysate ( Fig. 2d ). These bands were excised and analysed by liquid chromatography–tandem mass spectrometry (LC–MS/MS). The resulting data were searched against the Uniprot mouse proteome database appended with the FARP1 (F8VPU2) intron sequence that was identified as a translation product in the global proteomics experiment. The novel peptides from the presumed intron were identified in three of the bands as indicated in Fig. 2d . This extensive validation using IP and MS suggests that the bands observed in the WB do indeed contain various splice variants of FARP1, some of which include the novel intron. Furthermore, the fragmentation pattern of one of the novel peptides identified for FARP1 ( Fig. 2e ) matches that of its synthetic peptide. Taken together, the transcriptional and translational evidence suggests that this novel intron region is part of a larger unannotated variant of FARP1. The WB validation lends support to the genome-wide strategy for discovering novel non-canonical translation events. To predict the functional consequences of this large novel intron in the FARP1 protein, a disorder prediction analysis ( http://iupred.enzim.hu ) and domain mapping (SMART) were carried out. These analyses predicted a highly disordered region for this novel intron, and domain mapping using ELM ( http://elm.eu.org ) indicated numerous regulatory regions in this novel intron sequence when compared with the whole sequence. Figure 2f illustrates the quantitative estimation of a subset of regulatory regions that is enriched in the novel intron as compared with the entire protein sequence, suggesting that this region is possibly a hotspot for regulation by post-translational modifications. In addition, ribosomal footprinting data and RNA-seq data from HeLa cells provide further support for the expression of this FARP1 intron ( Supplementary Fig. 4 ). Mapping of novel peptides to genomic regions The novel peptides were mapped to their genomic origins and compared with existing annotations and the RNA-seq data. These comparisons led to a categorization of the novel peptides into five subgroups ( Fig. 3 ). Forty-nine of the novel peptides belonged to the set of peptides identified in the BLASTP search or were derived from 5′ leader sequences or 3′ end regions (group 1). A second group comprised 31 peptides that mapped to annotated pseudogenes (group 2). Ten of the peptides in this group were also identified in the BLASTP search as having computational evidence suggesting protein-coding potential. This result is consistent with previous studies showing that pseudogenes can be translated [19] ( Supplementary Fig. 5 ). A third group (group 3) included 79 peptides that mapped onto introns. These examples may reflect the existence of unannotated exons or intron inclusion events. One such example is the FARP1 locus discussed above. A particularly intriguing and unexpected group of 66 peptides (group 4) mapped onto the reverse strand from ( n =63) or near ( n =3) known exons and introns in protein-coding genes. Three of the peptides were found in the region upstream of the promoter, suggesting that they are derived from upstream antisense RNAs [8] in mouse cortical neurons [16] . One example is Flnb ( Supplementary Fig. 6 ), which shows evidence of a ~5-kb-long antisense transcript based on our RNA-seq data as well as RNA-seq data in both the mouse liver and kidney [20] . 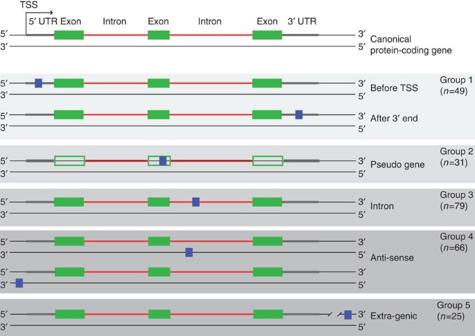Figure 3: Classification of novel peptides based on their genomic location. The top panel depicts the two DNA strands of a canonical protein-coding gene with exons (green boxes), introns (red lines) and the transcribed sequences before the first exon and after the last exon (grey lines, here referred to as 5′UTR and 3′UTR). The 250 novel peptides were divided into five groups based on their location relative to known genes. The peptide location is denoted here by blue boxes. The number of peptides in each group is indicated. In the last group (extragenic), the line is cut to indicate that there is a large distance (>10 kb) from the protein-coding gene. TSS, transcription start site. To validate the expression levels of a subset of identified ‘hit’ transcripts, total RNA was isolated, tested for its integrity and reverse transcribed ( Supplementary Table 3 ; Supplementary Fig. 7A ). Sequence verification confirmed the presence of the targeted antisense transcripts ( Supplementary Fig. 7B ). One of the novel peptides’ antisense to Cox17 (IILMPSLPAR), located on chromosome 16 overlapping but antisense to its second intron, was validated by synthetic peptide validation as discussed above ( Supplementary Fig. 7C ). All of the novel peptide groups described above were located within or in the vicinity of known protein-coding genes. Finally, a second unexpected set consisted of 25 peptides that mapped onto extragenic regions removed from any known protein-coding gene was found (group 5). Three of these peptides were also found in the ribosomal footprinting data [14] . Figure 3: Classification of novel peptides based on their genomic location. The top panel depicts the two DNA strands of a canonical protein-coding gene with exons (green boxes), introns (red lines) and the transcribed sequences before the first exon and after the last exon (grey lines, here referred to as 5′UTR and 3′UTR). The 250 novel peptides were divided into five groups based on their location relative to known genes. The peptide location is denoted here by blue boxes. The number of peptides in each group is indicated. In the last group (extragenic), the line is cut to indicate that there is a large distance (>10 kb) from the protein-coding gene. TSS, transcription start site. Full size image Quantitative analysis of the novel peptides Having determined the genomic context of the novel peptides, we set out to determine whether they were physiologically regulated in response to enhanced neuronal activity. Neuronal activation induces a gene expression programme involving several hundred genes as well as ncRNAs [5] . In the experimental set-up ( Fig. 1 ), mouse cortical neurons were stimulated using KCl, and tandem mass tags (TMT) labelling were used to quantify the relative abundance of each peptide at different time points following KCl stimulation. For each TMT channel, the same amount of protein, 100 μg, was used, and labelling bias was tested by assessing the median of log 2 intensities from all the channels ( Supplementary Fig. 8 ). The medians across the channels had a s.d. of 0.16 and a coefficient of variance of 0.02. This suggests that there is no inherent mixing irregularities in the total pool of labelled sample, and the differential peptide abundances observed among time points are true observations and hence could be biologically relevant. In addition, TMT labelling efficiency was evaluated to be 99.5% of all unique and high-confidence peptides, of which 98.3% are fully labelled (labelled on amino-terminal and internal lysine residues) with TMT reporter ions indicating that there is no significant loss of peptides that would affect quantitation. All the above validations highlight our careful and comprehensive assessment of the quantitative changes of the novel peptides and hence indicate that the abundances of the known proteins ( Supplementary Fig. 9 ) and novel peptides ( Fig. 4 ) are modulated by KCl depolarization. 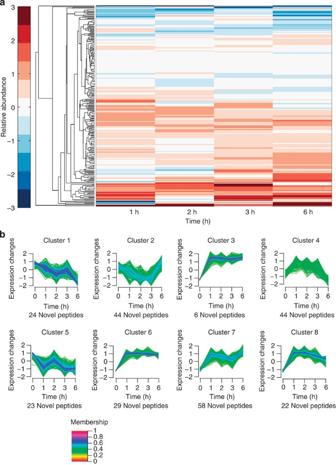Figure 4: Quantitative regulation of novel peptides. (a) Hierarchical clustering of the relative abundance temporal profiles for novel peptides (250 peptides). Each row represents one peptide. The four columns indicate abundance at 1, 2, 3 and 6 h post KCl stimulation. The colours represent up- or downregulation with respect to the 0 h time point (see colour map on left, a.u.). The clustering reveals several distinct regulatory patterns present both for known and novel peptides. These regulatory patterns are similar to those shown for known proteins inSupplementary Fig. 8. (b) Clusters of both known proteins and novel peptides showing similar temporal regulation post KCl stimulation. The numbers of novel peptides in each cluster are indicated. The membership scale reflects how well the regulation of a protein matches the consensus profile. Figure 4: Quantitative regulation of novel peptides. ( a ) Hierarchical clustering of the relative abundance temporal profiles for novel peptides (250 peptides). Each row represents one peptide. The four columns indicate abundance at 1, 2, 3 and 6 h post KCl stimulation. The colours represent up- or downregulation with respect to the 0 h time point (see colour map on left, a.u.). The clustering reveals several distinct regulatory patterns present both for known and novel peptides. These regulatory patterns are similar to those shown for known proteins in Supplementary Fig. 8 . ( b ) Clusters of both known proteins and novel peptides showing similar temporal regulation post KCl stimulation. The numbers of novel peptides in each cluster are indicated. The membership scale reflects how well the regulation of a protein matches the consensus profile. Full size image To identify patterns of co-regulation between the known proteins and novel peptides, the known protein abundance changes along with the novel peptide abundance changes were clustered together in an unbiased way using GProX (version 1.1.12) software. Results of the clustering analysis indicate that eight clusters identify discerning patterns of co-regulation of known proteins and novel peptides ( Fig. 4b ). The number of novel peptides in each of the clusters is listed in Fig. 4b . Extrapolating from this data and from our own previous analyses [21] , [22] , it can be predicted that these novel peptides are co-regulated in similar manner as the known proteins in each of the clusters. Some of the known proteins include CamKIId, Gria1 and Shank2, which are known to be temporally regulated with KCl stimulation in neurons. Using a custom unprocessed transcriptome database from the same experimental context as reported here for the unbiased examination of the proteome is a robust means to identify the existence of peptides derived from regions classified as noncoding throughout the genome. Although it is possible that some of these non-canonical peptides are the result of biological noise, this interpretation would require ‘errors’ at multiple levels, including transcriptional sloppiness by RNA polymerase, followed by the stable survival of non-polyA transcripts, export of these species into the cytoplasm, recognition by the ribosomal machinery and translation. The consistency of the findings, which are derived from pooling large numbers of cells, together with the validation, cast doubt on an interpretation purely based on biological noise. Instead, the discovery of non-canonical translation products and the validation of 250 novel peptides are consistent with several different lines of evidence, including ribosomal profiling studies [14] , characterization of short open-reading frames [19] , [23] , [24] , [25] and studies examining translation of pseudogenes [26] , which have pointed to a more extensive proteome than what is described by current databases. Most MS analyses, including the one presented here, are not saturating, and the number of detected protein products is much lower than the number of mRNAs detected by RNA-seq. Our RNA-seq data identified ~12,000 transcripts corresponding to canonical protein sequences, the proteomics data gave evidence for ~25% of the canonical transcripts. Extrapolating from this observation, it can be estimated that at least four times as many novel peptides are yet to be discovered under the current experimental conditions. Furthermore, it can be speculated that examining other tissues and biological conditions will uncover an even richer set of non-canonical translational events. The biological function, if any, of the novel peptides described here is not known. Several studies have suggested that evolutionarily conserved regions are more likely to be functionally important. Sequence conservation for the 250 novel peptides was investigated in 28 vertebrate species using the MultiZ alignment [27] . The results show that there are 30 peptides with significant evidence of purifying selection ( Supplementary Table 1 ) and that the translated sequences found in many species are more likely to show evidence of purifying selection ( Supplementary Fig. 10 ), consistent with studies of protogenes in yeast [28] . The observation that peptides derived from non-canonical translational events show dynamic regulatory patterns under physiological conditions similar to those characterized for well-established proteins further suggests the possibility that these peptides may also play functional roles. Future examination of other tissues and conditions combined with functional studies will shed light on the biological roles of the uncharted proteome. Brief overview of the experimental design and MS analysis Neuronal cultures were grown and depolarized with KCl for 0, 1, 2, 3 and 6 h (three biological repeat experiments were performed independently). Proteins were extracted and digested into peptides from neuronal cell lysates of each time point. Peptides from the five time points in each experiment were labelled with five different isobaric MS labels as follows: TMT-127 for 0 h, TMT-128 for 1 h, TMT-129 for 2 h, TMT-130 for 3 h and TMT-131 for 6 h (TMT-126 was used to label pre-stimulated neurons). After labelling, the peptides were pooled together and separated based on their isoelectric point differences into 24 fractions. Hence, a total of 24 × 3=72 fractions were collected and analysed by MS. Each sample was analysed three times by LC–MS/MS (at least three technical repeats were performed resulting in 238 MS raw data files), with a few re-analysed. These 238 files were grouped and then searched against mouse database. Unmatched peptides to the mouse database were then exported and searched against the custom RNA-seq database in six frames. After stringent filtering of the results, peptides designated as novel peptides were further validated by computational and biochemical methods including synthetic peptide matching, RT–PCR, WB, IP confirmed by MS and bioinformatics analysis. Each experiment is described in detail below. Animals All experimental procedures were performed in compliance with animal protocols approved by the IACUC at Children’s Hospital Boston, Boston, MA. We used embryos at age embryonic day (E) 16 from the C57BL6 mouse strain for neuronal cultures. Mouse cortical cultures Cortices of the mice embryos (C57BL/6, Charles River) at stage E16.5 were dissected and dissociated in 1 × Hank’s Balanced Salt Solution (HBSS; 14175-046, Life Technologies), 100 mM MgCl 2 , 10 mM kynurenic acid, 100 mM HEPES, 20 mg ml −1 trypsin (LS003736, Worthington Biochemicals) and 0.32 mg ml −1 L -cysteine (C7352, Sigma) for 10 min. Trypsin treatment to dissociate cells was terminated with three 2 min washes in 1 × HBSS with 10 mg ml −1 trypsin inhibitor (T6522, Sigma). Cells were triturated with a flame-narrowed Pasteur pipette for complete dissociation. Neurons were seeded at an approximate density of 4 × 10 7 on 15 cm dishes. The dishes were pre-coated overnight with 30 μg ml −1 poly-ornithine (P8638, Sigma) in water, washed three times with autoclaved water and washed once with Neurobasal Medium (21103049, Life Technologies) before use. Neurons were maintained in 30 ml filtered Neurobasal Medium containing 1 M glucose, B27 supplement (17504-044, Invitrogen), penicillin–streptomycin (50 μg ml −1 penicillin, 50 U ml −1 streptomycin; P0781, Sigma) and 1 mM glutamine (G6392, Sigma). Neurons were grown in vitro for 7 days. Eight millilitre of the medium was replaced with 10 ml fresh warm medium on the 4th and 6th days. KCl depolarization of neurons Neuronal cultures at day 6 were treated overnight with 1 μM tetrodotoxin (1078, Tocris) and 100 μM D (−)-2-amino-5phosphonopentanoic acid (D-AP5; 0106, Tocris) and cells were collected at 0, 1, 2, 3 or 6 h after incubation with 55 mM KCl in culture media. TMT labelling and peptide fractionation Cells were lysed on ice for 10 min using lysis buffer (50 mM Tris–HCl, pH 7.4, 150 mM NaCl, 1% NP-40, 1 mM phenylmethylsulphonyl fluoride) containing protease inhibitors (Roche complete protease inhibitor cocktail tablets) and phosphatase inhibitors (Sigma phosphatase inhibitor cocktails I and II). Cells were passed through a 27G needle multiple times, sonicated briefly and centrifuged for 30 min, 4 °C at 20,000 g to clear the solution. Clear lysates were collected, transferred to new tubes and protein concentrations estimated using a BCA assay kit (23225, Thermo Scientific). Protein precipitation and digestion were carried out as described by Winter et al. [29] Briefly, 100 μg of protein was precipitated from each time point using 1 ml of ice-cold chloroform/methanol. The pellets were re-dissolved in 0.1% Rapigest (186001861, Waters) in 100 mM TEAB (triethyl ammonium bicarbonate; 17902, Sigma) and incubated at 37 °C for 15 min. Trypsin (V5280, Promega) was added to the samples and incubated at 37 °C for 45 min to dissolve the pellet. Samples were reduced with 20 mM dithiothreitol (DTT) for 60 min at 56 °C and alkylated with 1% acrylamide for 45 min at room temperature (RT). Further trypsin was added to a final enzyme to protein ratio of 1:100 and the mixture was incubated at 37 °C overnight. Peptide samples from each time point were acidified using 5 μl trifluoroacetic acid and incubated for 45 min at 37 °C to precipitate the RapiGest followed by centrifugation for 30 min at 20,000 g . Clear supernatants were desalted using Oasis HLB cartridges (186006339, Waters). Briefly, the columns were washed twice with 70% acetonitrile (ACN) 0.1% formic acid (FA) and twice with 0.1% FA. The sample pool was passed twice through each individual column, washed four times with 0.1% FA and eluted twice with 30% ACN 0.1% FA, twice with 50% ACN 0.1% FA and twice with 70% ACN 0.1% FA. Individual eluate fractions were pooled and samples dried in a vacuum centrifuge. Dried samples were resuspended in 0.1 M TEAB and peptide concentrations quantified using the BCA assay. For each sample, peptides from different time points after KCl stimulation were labelled with one of the five TMT labels (PI-90064, Thermo Fischer Scientific) for 3 h at RT following the manufacturer’s protocol. The samples were combined, partially dried using a vacuum centrifuge and desalted using Oasis HLB cartridges as described above. The dried peptides were resuspended in ampholyte solution (pI 3–10) and fractionated overnight into 24 fractions based on their isoelectric point using an OFFGEL fractionator (Agilent) according to the manufacturer’s instructions. The fractions were desalted and analysed using LC–MS/MS. MS analysis Peptide samples were loaded directly onto an in-house-packed reverse phase column using 5 μm, 200 Å particles (magic C18, Michrom) and PicoTip Emmiters (New Objective) with an autosampler/nanoLC set-up (2D nanoLC, Eksigent) at a flow rate of 1 μl min −1 . After loading, the column was washed for 5 min at 1 μl min −1 with 99%A (water with 0.2% FA) 1%B (acetonitrile with 0.2% FA) followed by elution with a linear gradient from 1% B to 35% B at 400 nl min −1 in 60 min. Peptides eluting from the column were ionized in the positive-ion mode and the six most abundant ions were fragmented in the pulsed-Q Dissociation (PQD) mode [30] to allow for the detection of low-mass-range reporter ions. Briefly, the LTQ-Orbitrap was run in positive-ion mode. Full scans were carried out with a scan range of 395 to 1,200 m / z . Normalized collision energy of 35 was used to activate both the reporter ions and parent ions for fragmentation. Scans were carried out with an activation time of 30 ms. The isolation window was set to 1.0 m / z . Testing labelling efficiency For each of the TMT channels, equal amounts of protein, 100 μg, were used. Labelling bias was tested by assessing the log 2 intensities from all the channels ( Supplementary Fig. 8 ). The median across the channels had a s.d. of 0.16 and a coefficient of variance of 0.02, suggesting that there is no inherent mixing irregularities in total pool of labelled sample and the differential peptide abundances observed among time points are true observations. In addition, TMT labelling efficiency was evaluated to be 99.5% of all unique and high-confidence peptides, of which 98.3% are fully labelled (labelled on N terminal and internal lysine residues) with TMT reporter ions. The labelling efficiency of fully labelled peptides and the median intensities calculated for each channel indicate that there is no quantitative bias that would affect the results reported in the profile data. MS data analysis The proprietary Thermo Scientific .raw files (238 in total as explained above) were converted into six .mgf files and MS/MS data was queried against the Uniprot February 2012 (canonical and isoform sequences) protein sequence database, containing common contaminations and concatenated to its decoy version, using Mascot v2.3 (Matrix Science). TMT peptides were searched with enzyme specificity trypsin, two missed cleavage sites, carbamidomethyl (Cys), oxidation (Met), deamidation (N), and Gln to pyro Glu (N-terminal Q) and phosphorylations on S/T/Y and TMT-6plex (N termini and Lys) as variable modifications. Only 226,471 (20%) of the spectra were matched to the mouse database, resulting in 15,516 peptides that were unique. They were grouped into 3,284 proteins with a 1% protein FDR cut-off for proteins and at least two peptides per protein were identified. This corresponded to a Mascot cut-off score of 26.93 and above for each protein. The remaining 904,922 (80%) unmatched spectra were exported and searched against a custom database generated from RNA-seq data comprising all the transcribed regions [16] . The nucleotide database was concatenated to common contaminants and its decoy version and searched using Mascot v2.3 in all six frames with the following parameters: enzyme specificity trypsin, two missed cleavage sites, carbamidomethyl (Cys), oxidation (Met), deamidation (N), and Gln to pyro Glu (N-terminal Q) and TMT-6plex (N termini and Lys) as static modifications. A stringent 1% local FDR was used to select for high-confidence-matched spectra, resulting in 7,722 matched spectra (PSMs). To further ensure that only high-quality matches were included, only the 1,584 matched spectra with an expectation value <0.05 were chosen for further analysis. The expectation value is calculated by the search engine (Mascot v2.3), and it is equivalent to the E -value in a BLAST search. In total, there were 250 distinct peptides that mapped uniquely to the mouse genome and did not overlap with the 3,284 proteins. This set of high-confidence-unmatched peptides that are matched to experimentally defined nominally noncoding transcripts is referred to as novel peptides. Synthetic peptide labelling and validation Synthetic peptides (JPT Peptide Technologies) were dissolved as per instruction. These peptides were pooled in equimolar concentration and categorized into six groups. Each peptide group was mixed with one of the six TMT labels (Thermo Scientific) for 3 h at RT. The reactions were quenched with 5% hydroxylamine in 100 mM TEAB and incubated for 15 min at RT. The samples were desalted with micro spin Silica C18 columns (Nest Group) following manufacture’s guidelines. Briefly, the columns were washed twice with 70% ACN (with 0.1% FA) and washed twice with 0.1% FA. The sample pool was passed twice through each individual column, washed four times with 0.1% FA and eluted twice with 30% ACN (with 0.1% FA), twice with 50% ACN (with 0.1% FA) and twice with 70% ACN (with 0.1% FA). The eluted fractions of each individual pool were combined and dried in a speed-vac (Thermo Scientific) at RT. The pellet was re-dissolved in 5% ACN (with 5% FA) loading buffer and analysed on four different instruments: a Q-Exactive (Thermo scientific) and on three instruments capable of PQD—an Orbitrap Elite (Thermo scientific) and two Orbitrap Velos at Beth Israel and Deaconess Medical Center and at the University of Bonn (Thermo scientific). The .raw files were searched against the custom RNA-seq database. The spectra and the fragmentation pattern for each of the synthetic peptides were compared and validated to the ones from the experiment, denoted as ‘identified’. Briefly, the top 90% matched fragment ions were compared between the synthetic peptide spectra and identified peptide spectra using Spearman rank-order correlation analysis. All the correlations were checked for a significant P value of 0.05 or less and positive correlation coefficient for all the instrument types. Finally, the matched y and b ions indicated by their respective fragmentation tables were also mapped. RT–PCR validation Total RNA isolation for RT–PCR validation was done using mirVana isolation kit (AM1560, Ambion). We collected and combined 0, 1, 2, 3 and 6 h post-KCl stimulation time points for cortical neuron cultures that were plated in equal density. Cells were washed with phosphate-buffered saline, lysed on ice with vortexing in lysis/binding solution as per the manufacturer’s instruction. The lysate was treated with 1/10 volume of miRNA homogenate additive for 10 min on ice and was organically extracted with acid-phenol:chloroform mixture. The aqueous phase was recovered and mixed with 1.25 volumes of 100% ethanol. The mixture was further purified through filter cartridge, washed and eluted with nuclease-free water. The RNA eluate was analysed (Agilent 2100 bioanalyzer nano series) to determine high-quality, intact RNA without DNA contamination and concentration was determined using a nanodrop spectrophotometer ( Supplementary Fig. 7A ). First-strand cDNA was synthesized using SuperScript First-Strand synthesis system (11904-018, Invitrogen). Briefly, total RNA sample was incubated with random hexamer primers to include all RNA for cDNA synthesis and dNTP mix at 65 °C for 5 min, then placed on ice for 1 min. The sample was mixed with 2 × reaction mix of reverse transcription buffer, MgCl 2 , DTT and RNAaseOUT and incubated at RT for 10 min, then incubated at 42 °C for 50 min. The reaction was terminated by heating at 70 °C for 15 min, then on ice. To ensure the sensitivity of PCR, the cDNA–RNA hybrid molecule was treated with RNase H at 37 °C for 20 min. The cDNA was then used to amplify specific novel regions of selected length containing peptide match regions identified using the mass spectra and deep-sequencing data. Primers were synthesized with IDT custom oligo, designed using OligoPerfect designer (Invitrogen) and Tm was optimized using Finnzyme calculator (Thermo Scientific). Supplementary Table 3 lists the regions of interest and primer sequences. PCR was performed using Phusion HF buffer, dNTPs mix and Phusion hot start DNA polymerase with initial denaturation at 98 °C for 30 s, denaturation at 98 °C for 10 s, annealing at Tm of the lower tm primer (for 20 nucleotides or less) and 3 °C higher than the Tm of lower tm primer (for more than 20 nucleotides) for 30 s, extension at 72 °C for 30 s per kb template length and 30 cycles. Final extension was done at 72 °C for 10 min, followed by 4 °C. The PCR products were run on 1% agarose with ethidium bromide in 1 × buffer solution containing a mixture of Tris base, acetic acid and EDTA (TAE) buffer ( Fig. 2c ; Supplementary Fig. 6B ). Products were gel purified using QIAQuick PCR purification columns (28104, Qiagen) and sequenced conventionally. The results were mapped to the template region using the ClustalW2 (EMBL-EBI) tool and translated into six frames using ExPASy tool to validate for peptides match. FARP1 IP and WB analysis Whole-brain tissue was lysed in buffer (50 mM Tris–HCl, pH 8, 150 mM NaCl, 1% NP-40, 0.5% sodium deoxycholate, 0.1% SDS, 0.004% sodium azide, protease inhibitor tablet) using bead beater homogenizer (Precellys) for 6,800 r.p.m., 3 × 15 s with 60 s rest cycle. The lysate was centrifuged at 14,000 r.p.m., 10 min at 4 °C. FARP1 antibodies K-20 (sc-74927, 2 μg per 500 μg of lysate for IP, 1:500 for WB, Santa Cruz Biotechnology) and FARP1 H-300 (sc-98722, 2 μg per 500 μg of lysate for IP, 1:500 for WB, Santa Cruz Biotechnology) were tested separately for IP and incubated with lysate for 2 h. The immuno-complexes were pulled down using protein A/G agarose beads (Santa Cruz Biotechnology) in an overnight incubation with rotation. The beads were pre-blocked with bovine serum albumin to reduce nonspecific immunoglobulin binding. The immune precipitates were sedimented at 1,000 g , 5 min at 4 °C. The beads were washed four times with RIPA buffer containing 150 mM salt. The beads were resuspended in Laemmli buffer containing β-mercaptoethanol and boiled for 3–4 min. The lysate and IP eluate samples were run on 4–12% SDS–PAGE gel (NP0335BOX, Invitrogen) and were subjected to WB analysis using the FARP1 primary antibody K-20 (sc-74927) as a probe in dilutions described above. A secondary goat antirabbit IgG-HRP antibody (sc-2054, 1:5,000 dilution) was then used for the WB (Santa Cruz Biotechnology). WB was developed by Super Signal West Pico chemiluminescence kit (34080, Pierce). The Coomassie-stained gel bands were analysed by MS/MS. The peptides were extracted, reduced with DTT, alkylated with iodoacetamide and digested with trypsin before running on a QE instrument with a 60-min gradient to acquire a base peak chromatogram intensity of e 9 – e 10 . The raw files were converted into .mgf files and searched using mouse proteome database (Uniprot February 2012 (canonical and isoform sequences) protein sequence database) containing common contaminations and concatenated to its decoy version, using Mascot v2.3 (Matrix Science) appended with mouse FARP1 Uniprot identifiers and intron region (983 bases) in coding frame using ProteinPilot search engine software v4.5.1. The data was analysed to identify peptides from FARP1. Bioinformatics analysis Each of the 250 peptides reported in Supplementary Table 1 were inspected manually using the UCSC Genome browser. In addition to using the chromatin IP sequencing (ChIP-Seq) and RNA-Seq data from mouse neurons, the RNA-Seq data from the mouse ENCODE was also used [20] . The initial assignment into different categories was carried out by an algorithm, and the assignment was based on the location of the transcribed region and peptide relative to known genomic features. In some cases, the category was changed following the manual inspection. Clustering of novel peptides and known proteins The intensities for each peptide were normalized by dividing the values at 1, 2, 3 and 6 h by the value at 0 h. Next we carried out unsupervised hierarchical clustering of the log 2 values for the temporal profiles using Matlab’s ‘clustergram’ function. The clustering was based on the Euclidean distance between the intensity profiles and the same settings were used for the known ( Supplementary Fig. 9 ) and the novel peptides ( Fig. 4a ). Co-clustering of novel peptides and known proteins To identify patterns of co-regulation between the known proteins and novel peptides, the known protein abundance changes along with the novel peptide abundance changes were clustered together in an unbiased way using GProX (version 1.1.12) software. Results of the clustering analysis indicate that eight clusters identify discerning patterns of co-regulation of known proteins and novel peptides ( Fig. 4b ). The number of novel peptides in each of the clusters is listed in Fig. 4b . All ratios in each experiment were standardized before clustering (the mean was deducted from the values and divided by their s.d.). The membership scale reflects how well the regulation of a protein matches the consensus profile. Ribosomal footprinting analysis Ribosomal footprinting data for elongating ribosomes for mouse embryonic stem cells was downloaded from gwips.ucc.ie. To identify peptides with significant levels of ribosomal footprinting reads, the peptide positions were first converted to mm10 coordinates, and then all peptides with five or more reads within 200 bp were extracted. On the basis of manual inspection in the genome browser at gwips.ucc.ie, 34 loci were determined to have evidence of ribosomal interactions. Phylogenetic comparison The MultiZ alignment for 28 species relative to mm9 was downloaded from the UCSC website. Around 142 peptides were found in alignment blocks by MultiZ, and the orthologous sequences for all other species that aligned to the same block were extracted. For each aligned peptide, the codons with one substitution were classified as either synonymous (S) or non-synonymous (N), and the total number of synonymous (dS) and non-synonymous (dN) events were recorded. For each peptide, the ratio dN/dS were calculated ( Supplementary Fig. 10 ) and a value <1 is characteristic of purifying selection. As a control, for each peptide, a sequence of the same length starting 1,000 bp downstream was extracted. Since only a few annotated exons in the mouse genome are longer than 1 kb, it is highly unlikely that the control sequences will be part of the same exon as the novel peptide. Thus, there is only a one-third chance that the control sequence will be in frame. To compensate for the fact that the frame of the controls is not known, the sequences starting 1,001 and 1,002 bp downstream were also extracted, and for each codon, the frame with the lowest dN/dS ratio was selected. This strict control did not have as many codons with dN/dS<1 as the data ( Supplementary Fig. 10 ), suggesting that the differences between the data and the control are real. To determine the threshold for when dN/dS is significant, the largest value where the number of peptides in the data is no longer at least 10 times larger than the control was chosen (the threshold chosen was 0.8). How to cite this article : Prabakaran, S. et al. Quantitative profiling of peptides from RNAs classified as noncoding. Nat. Commun. 5:5429 doi: 10.1038/ncomms6429 (2014). Accession codes: RNA-seq data is already published [5] , [16] . The data can be found on GEO with the code GSE21161 .